From chaos to selective ordering of vortex cores in interacting mesomagnets A spin vortex consists of an in-plane curling magnetization and a small core region (~10 nm) with out-of-plane magnetization. An oscillating field or current induce gyrotropic precession of the spin vortex. Dipole–dipole and exchange coupling between the interacting vortices may lead to excitation of collective modes whose frequencies depend on the core polarities. Here we demonstrate an effective method for controlling the relative core polarities in a model system of overlapping Ni 80 Fe 20 dots. This is achieved by driving the system to a chaotic regime of continuous core reversals and subsequently relaxing the cores to steady-state motion. It is shown that any particular core polarity combination (and therefore the spectral response of the entire system) can be deterministically preselected by tuning the excitation frequency or external magnetic field. We anticipate that this work would benefit the future development of magnonic crystals, spin–torque oscillators, magnetic storage and logic elements. Vortices are observed in the statics and dynamics of a variety of physical systems, such as fluids and plasma [1] , optics [2] , superconductors [3] and magnetic materials [4] . In patterned mesoscopic ferromagnets, the ground state of the static magnetization can have a form of a vortex that consists of a large region of in-plane curling magnetization (clockwise or anticlockwise sense of rotation or chirality) and a small core region (~10 nm) with out-of-plane magnetization, which can be pointing either up (+1) or down (−1) (positive or negative core polarity p ). When the vortex core is perturbed from its equilibrium state by an in-plane oscillating field or current, it begins a rotational (gyrotropic) oscillation with a characteristic eigenfrequency in the subgigahertz range [5] , [6] , [7] . In a magnetic dot that has a single vortex-state, the eigenfrequency of the gyrotropic oscillations of the vortex core for both directions of the core polarity ( p =±1) is the same. By contrast, in an array of coupled elements, the dynamic dipolar interaction eliminates this frequency degeneracy and results in collective gyrotropic excitations with different eigenfrequencies that depend on both the relative polarities and chiralities of the individual vortices [8] , [9] , [10] , [11] . An array of interacting magnetic dots form a vortex magnonic crystal [12] , [13] , similar to the case of coupled, uniformly magnetized elements [14] , [15] . The system can have a dynamically reconfigurable ground state characterized by different relative polarities and chiralities of the individual dots; and it can have a corresponding dynamically controlled spectrum of collective excitation modes that determine the microwave absorption of the crystal. The development of effective methods for dynamic control of the ground state in vortex-type magnonic crystals is fundamentally interesting and could also be important for possible microwave applications. Vortex chirality has been controlled in confined geometries using various techniques [16] , [17] . Manipulation of the vortex core polarity has been shown in individual elements by resonant in-plane [18] , [19] and perpendicular magnetic fields [20] , rotating magnetic fields [21] , pulsed currents [22] and spin-polarized currents [23] . However, control of the vortex core polarities in interacting vortex-state magnetic dots remains a challenge. In this work, we demonstrate an effective method for controlling the relative vortex core polarities in a model system of connected (slightly overlapping) vortex-state permalloy (Ni 80 Fe 20 ) magnetic dots. This method also permits the effective selection of a specific dynamic mode of microwave absorption. We utilize the geometry of connected double-dot structures because they have the potential to form building blocks of vortex magnonic crystals [12] , [13] . An advantage of the double-dot overlap structure is the strong dynamic interaction between the vortex cores and, consequently, the large difference between the eigenfrequencies of the gyrotropic dynamic modes that correspond to the same and opposite orientations of the interacting cores. In the remanent state of this structure, the configurations with the same ( p 1 p 2 =+1) or opposite ( p 1 p 2 =−1) core polarities are equally probable. Therefore, the selection of a particular dynamic mode in this system is achieved by first driving the system into a chaotic regime of continuous vortex core reversals via a large-amplitude external driving signal that has the same frequency as one of the dynamic gyrotropic modes of the system. Then, the driving amplitude is reduced so that the system relaxes to the state corresponding to the other collective gyrotropic mode that has a different eigenfrequency; therefore, the system can no longer resonantly absorb energy from the driving signal. Sample structure and measurement setup Permalloy (Ni 80 Fe 20 ) double-dot structures with dimensions of 2 × 1 × 0.048 μm 3 and vertical contact length of 740 nm were fabricated on top of shorted coplanar waveguide (CPW). Representative atomic force microscopy image for a dot pair is shown in Fig. 1a . The signal line of the CPW consists of >1,000 of such dot-pairs. Microwave measurements were performed in reflection mode using a vector network analyser as the current source. 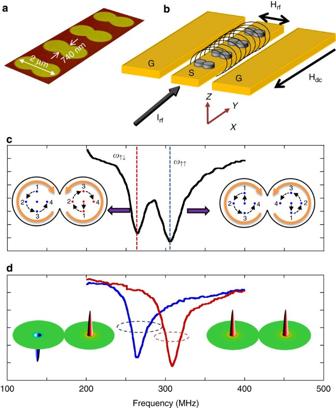Figure 1: Absorption spectra before and after mode selection. (a) Atomic force microscopy image of the connected double-disk structure with dimensions of 2 × 1 μm2. (b) Schematic of the CPW with connected double disks. (c) Absorption spectrum obtained at zero magnetic field with two absorption peaks corresponding top1p2=−1 and +1 at 265 and 305 MHz, respectively. The vortex core gyration in each disk is also illustrated. The solid line illustrates the chirality of the in-plane magnetization. The dashed lines define the direction of vortex core trajectories. (d) Absorption spectra obtained after high RF-amplitude treatment at fixed frequencies ofω↑↓(red curve) andω↑↑(blue curve). The insets show the resultant vortex core polarity combination in the disks. Figure 1b shows the schematic of the CPW, where the radio frequency (RF) field is applied along the long axis of the system ( x axis). The absorption spectrum for the as-grown sample at remanence for −15 dBm of input microwave power ( P Low ) is shown in Fig. 1c . This system of two vortex cores has an equal probability of having either of the two polarization combinations [24] . The two absorption peaks in Fig. 1c correspond to opposite ( p 1 p 2 =−1) and same ( p 1 p 2 =+1) polarity combinations. It should be noted that the measured spectra is the response from >1,000 dot pairs on the waveguide. As the structures are fabricated using electron-beam lithography technique, we believe that the effect of size variation on the resonant frequencies of the coupled modes is within the line-width of each excited mode. The eigenfrequencies for the two polarity combinations are 265 MHz ( ω ↑↓ ) and 305 MHz ( ω ↑↑ ), respectively. This spectrum is similar to the response from an array of elliptical particles [24] . The structure of the collective gyrotropic modes follows from the symmetry of the double-dot system ( Supplementary Fig. S2 ). For the p 1 p 2 =−1 state, the two vortex cores gyrate out-of-phase with each other along the direction of RF excitation ( x -axis) and in-phase in the orthogonal direction ( y -axis). However, for the p 1 p 2 =+1 state, the two cores gyrate in-phase for both directions, as schematically illustrated in Fig. 1c . Because the chiralities of the two vortices in a double-dot system are always opposite to each other, the p 1 p 2 =−1 mode is linearly polarized (the net magnetic moment oscillates along x -axis), whereas the polarization of the p 1 p 2 =+1 mode is elliptical (the net oscillating magnetic moment has both x and y components). Figure 1: Absorption spectra before and after mode selection. ( a ) Atomic force microscopy image of the connected double-disk structure with dimensions of 2 × 1 μm 2 . ( b ) Schematic of the CPW with connected double disks. ( c ) Absorption spectrum obtained at zero magnetic field with two absorption peaks corresponding to p 1 p 2 =−1 and +1 at 265 and 305 MHz, respectively. The vortex core gyration in each disk is also illustrated. The solid line illustrates the chirality of the in-plane magnetization. The dashed lines define the direction of vortex core trajectories. ( d ) Absorption spectra obtained after high RF-amplitude treatment at fixed frequencies of ω ↑↓ (red curve) and ω ↑↑ (blue curve). The insets show the resultant vortex core polarity combination in the disks. Full size image Demonstration of polarity control To explore the phenomenon of vortex core reversal in coupled vortices, the double-dot structures were driven at a high microwave power of 10 dBm ( P High ) at the resonance frequency of one of the collective modes. When the power was subsequently reduced to a minimum accessible value of P Low , which was used to probe vortex excitations in the linear regime, only one absorption peak that corresponded to the second collective mode was observed in the frequency spectrum. This result indicates that when the system is excited by a large-amplitude signal at the frequency of ω ↑↓ , with the reduction of the driving amplitude, the system relaxes to the ground state of core polarities that correspond to the collective mode with the frequency of ω ↑↑ and vice versa. The representative absorption spectra for two different excitation frequencies of ω ↑↓ (red curve) and ω ↑↑ (blue curve) are shown in Fig. 1d . Indeed, only one absorption peak, corresponding to the collective mode that is non-resonant with the frequency of the driving signal, is present in each low-amplitude spectrum of the system. In the following, the excitation process of the vortex core motion with a large-amplitude external signal P High and the subsequent reduction of the signal amplitude to P Low at a constant driving frequency corresponding to one of the collective modes will be termed as the initialization procedure. The absorption spectra obtained after this procedure will be measured at P Low to identify the dynamic collective modes (corresponding to a particular combination of vortex polarities) present in the system. Micromagnetic modelling To simulate the experimental results, the gyrotropic motion of the vortex cores in the two dots were excited at a high RF amplitude of 52 Oe (sufficiently strong to induce the vortex core reversal), which was then gradually reduced to 2 Oe in steps of 0.1 Oe per cycle. 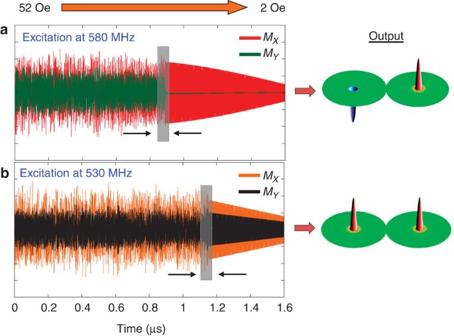Figure 2: Demonstration of mode selection using micromagnetic simulations. Micromagnetically simulated time evolution of the magnetizations in the connected double-disk structures at two different excitation frequencies of (a) 580 MHz and (b) 530 MHz, while varying the RF-amplitude from 52 to 2 Oe. The final output polarization state of the system is independent of the input combination (which can be either +1 or −1) and is only dependent on the excitation frequency. Figure 2 shows the time evolution of the average magnetization when the system was excited at ω ↑↑ ( Fig. 2a ) and ω ↑↓ ( Fig. 2b ). The initial combination of the vortex core polarities can be chosen either parallel or antiparallel. One can easily observe that at sufficiently high RF fields, the two vortex cores undergo continuous reversals, as seen from the chaotic and unsynchronized oscillations of magnetization. However, below a certain RF field, both the x and y components of the dot magnetization stabilize to steady-state oscillations corresponding to a polarity combination of the non-resonant mode. Importantly, this reveals that the resultant state of the system does not depend on the input ground state of vortex core polarities; it only depends on the initialization frequency. Therefore, the final configuration of the system is completely decoupled from the driving signal and cannot absorb energy from this signal. Figure 2: Demonstration of mode selection using micromagnetic simulations. Micromagnetically simulated time evolution of the magnetizations in the connected double-disk structures at two different excitation frequencies of ( a ) 580 MHz and ( b ) 530 MHz, while varying the RF-amplitude from 52 to 2 Oe. The final output polarization state of the system is independent of the input combination (which can be either +1 or −1) and is only dependent on the excitation frequency. Full size image The transition from chaotic to synchronized vortex core motion, marked as the shadow region in Fig. 2a , is of particular interest. This region (shadow area in Fig. 2b ) is presented in Fig. 3a . It has been established that the dynamically-driven core reversal is mediated by a series of complex processes: nucleation of a transient vortex–antivortex pair followed by the annihilation of the original vortex with the newly formed antivortex [18] , [23] . Apart from the critical velocity and critical radius defining the criteria for the core reversal, a well-defined threshold value of the exchange energy is also necessary for this process [25] . Therefore, to quantify the core reversal occurring in the interacting vortices, the exchange energy of the coupled system was considered and the graph of this energy is shown in Fig. 3a . Each peak in the exchange energy is associated with a vortex core reversal. Because the average magnetization response ( M X and M Y ) does not directly provide information about the core reversals in each dot, the magnetization components of each dot were separately deduced from the simulations. These components are shown in Fig. 3b , respectively. Surprisingly, we observed that in a particular period of time, only one core in the double-disk system undergoes reversal, whereas the other one performs a steady-state rotational motion. This result is surprising because the system is continuously driven using high oscillating fields and only one core undergoes several reversal processes. For instance, from t 1 =2–38 ns, the core in dot 2 undergoes continuous core reversals, whereas the core in dot 1 rotates with the same frequency as the driving frequency. The vortex core trajectories for this time span are shown in Fig. 3d . After ~38 ns, there is a transfer of energy between the cores, and the core in dot 1 begins to reverse. The respective core trajectories for this state are shown in Fig. 3e . The dot whose vortex core undergoes reversal is indicated by grey regions in Fig. 3b . This behaviour is remarkable because it demonstrates that a systematic reversal pattern exists even in a quasi-chaotic reversal regime (to investigate this phenomenon, an analytical approach was utilized; the detailed description of this approach is provided in Supplementary Discussion). It was observed that the relative phase difference between the two coupled modes determines the particular core that undergoes reversals. The dynamics induced due to this reversal process forces the phase difference to change its sign and consequently, the second core begins to reverse. This transfer process continues until the excitation amplitude is reduced. A particular core continues to reverse for a characteristic time T that is on the order of the inverse of the mode frequency difference, T ~1/Δ ω . 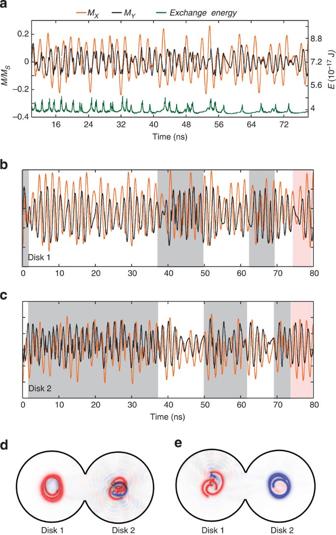Figure 3: Transition region between chaos and order. (a) Time-dependent average magnetization and exchange energy response of the transition region shown inFig. 2b. (b,c) The computed magnetization responses from individual disks. The grey region corresponds to the vortex core reversal in a particular disk. The vortex core trajectories in each disk when the vortex core reversal occurs in only one disk are shown indande. Presence of only one colour in a disk (either red or blue) indicates constant gyration of the vortex core (as shown in disk 1 ofdand disk 2 ofe). Vortex core reversal is marked by two colours in the disk for the original and reversed polarity of the core (disk 2 indand disk 1 ine). Figure 3: Transition region between chaos and order. ( a ) Time-dependent average magnetization and exchange energy response of the transition region shown in Fig. 2b . ( b , c ) The computed magnetization responses from individual disks. The grey region corresponds to the vortex core reversal in a particular disk. The vortex core trajectories in each disk when the vortex core reversal occurs in only one disk are shown in d and e . Presence of only one colour in a disk (either red or blue) indicates constant gyration of the vortex core (as shown in disk 1 of d and disk 2 of e ). Vortex core reversal is marked by two colours in the disk for the original and reversed polarity of the core (disk 2 in d and disk 1 in e ). Full size image An energy transfer mechanism was previously observed in separated dots by Jung et al. , [9] where the ground state of only one of the dots was perturbed by a pulsed RF field. This ground-state perturbation introduced an asymmetry in the initial conditions and, hence, the system behaved like coupled harmonic oscillators where the magnetic potential energy of a vortex core was transferred from one dot to the other. Therefore, the transfer of the vortex potential energy observed in our case for the chaotic regime (as opposed to the linear regime) is unique. When the amplitude of the driving signal is reduced, the number of vortex core reversal events decreases and the rotation of both vortex cores eventually become steady without any further reversals (pink region in Fig. 3b ). For the simulated responses shown in Fig. 3 , the structure was excited at a fixed driving frequency of 530 MHz, which is the resonance frequency of the p 1 p 2 =−1 mode. Therefore, for this driving frequency, the ground state with opposite polarities of the interacting vortex cores is more susceptible to the core reversal. By contrast, for the ground state with the same polarities of the vortex cores (and having a different eigenfrequency), a substantially larger driving amplitude is required to induce the vortex core reversal. This resonance asymmetry is responsible for our ability to select a particular dynamic collective mode (and a corresponding particular configuration of the vortex core polarities). As a result of the initialization process described above, after passing through a quasi-chaotic regime of continuous core reversals followed by a subsequent decrease of the driving amplitude, the system settles into a regime of steady-state vortex gyration with the mode whose eigenfrequency is non-resonant with the driving frequency. RF power dependence on polarity control In the experiments we applied a fixed high-amplitude driving signal of P High to induce the vortex core reversals. At the same time, the simulation results clearly indicate that there is a certain threshold in the driving power, below which the mode selection procedure does not work. To experimentally verify this, we subjected our double-dot samples to different amplitudes of driving fields. The experimentally measured colour-coded frequency spectra of the system subjected to the driving frequencies of ω ↑↓ =265 MHz and ω ↑↑ =305 MHz are summarized in Fig. 4a , respectively. To obtain these spectra, we varied the value of P high during the initialization process at fixed excitation frequencies of 265 and 305 MHz. Low-power frequency scans were then performed to identify the collective modes present in the system. The horizontal dotted lines indicate the critical driving amplitudes above which one of the collective modes in the system completely disappears. For example, in Fig. 4a , where the driving frequency is ω ↑↓ =265 MHz, a driving power of <−2 dBm is not sufficient to induce vortex core reversals and, consequently, both absorption peaks are present in the spectrum. However, for driving powers >−2 dBm, the excitation amplitude is sufficiently strong to induce the core reversal process and, consequently, only one collective mode (not resonant with the driving) is present. 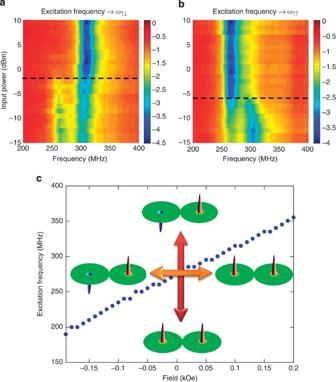Figure 4: Drive amplitude, frequency and magnetic field dependence on mode selection. Frequency spectrum obtained at −15 dBm (PLow) and 230 MHz for various high RF-amplitudes at constant excitation frequencies of (a) 264 MHz and (b) 304 MHz. The dashed lines inaandbcorrespond to the critical threshold magnitude of input power, which is required to completely suppress the resonant mode. (c) Universal phase diagram constructed for the excitation frequency versus external magnetic field. The circular dots mark the transition region where selecting a specific field direction (left→right or right→left) at a fixed excitation frequency will yield a desired polarity combination in the disks. Conversely, vertical arrows that the same polarity combination can also be chosen by keeping the magnitude of external magnetic field constant and sweeping the excitation frequency. Figure 4b (where the driving frequency is ω ↑↑ =305 MHz) shows the same effect, but with a different collective mode as the resultant ground state. The difference in the critical driving amplitudes (shown by dotted lines) for these two distinct cases is a direct measure of the strength of the dynamical interaction between the collective gyrotropic modes in our double-dot sample. Figure 4: Drive amplitude, frequency and magnetic field dependence on mode selection. Frequency spectrum obtained at −15 dBm ( P Low ) and 230 MHz for various high RF-amplitudes at constant excitation frequencies of ( a ) 264 MHz and ( b ) 304 MHz. The dashed lines in a and b correspond to the critical threshold magnitude of input power, which is required to completely suppress the resonant mode. ( c ) Universal phase diagram constructed for the excitation frequency versus external magnetic field. The circular dots mark the transition region where selecting a specific field direction (left→right or right→left) at a fixed excitation frequency will yield a desired polarity combination in the disks. Conversely, vertical arrows that the same polarity combination can also be chosen by keeping the magnitude of external magnetic field constant and sweeping the excitation frequency. Full size image Thus, two collective gyrotropic modes with substantially different frequencies were observed in the two-vortex model system. Our experiment clearly demonstrated that the final ground state of the system, which was achieved after the initialization process, is only dependent on the driving frequency and not on the initial ground state of the system (that is, the initial combination of the vortex core polarities). The mode that is present at the end of the process is non-resonant with the driving field, and it is consequently completely decoupled from the driving field. Dependence of resultant polarity combination on external magnetic field The frequencies of collective modes are strongly dependent on the external magnetic field. Consequently, varying the bias field can be used to tune the eigenfrequencies of the system. Thus, a particular collective mode can be coupled or decoupled to RF input signal of given (fixed) frequency by varying the strength of the external field when applied along the y axis of the system. This process is illustrated in Supplementary Fig. S1 , where a particular collective mode can be selected by choosing a proper field sweep range. On the basis of the universality of the mode selection phenomena, a phase diagram has been constructed with respect to the excitation frequency and the external magnetic field, as shown in Fig. 4c . This experimental phase diagram for the connected double-dot structure specifically provides the desired parameters for defining the ground state with either of the two polarity combinations. An external magnetic field can be swept horizontally on the phase diagram at a constant excitation frequency and, depending on the direction of the sweep and on the stop field, a unified state can be set in the entire array. Similarly, the frequency can be swept vertically in the presence of a constant magnetic field to obtain a specific ground state. We developed a new and effective method to control the ground state determined by the relative vortex core polarities and the dynamic excitation mode in a model system of coupled vortex-state magnetic dots. The method involves driving the system by a strong periodic driving field into a quasi-chaotic regime of continuous vortex core reversals. This process is followed by a gradual reduction of the driving field and relaxing of the system to a ground state, which supports the dynamical mode that is non-resonant with the driving frequency and is therefore non-responsive with the driving field. A similar approach can be used to dynamically select a particular ground state in a vortex-state magnonic crystal [12] , [13] and in other physical systems that have multiple stable ground states, such as arrays of coupled nano-oscillators [26] , [27] or spin-ice-type lattices [28] . Furthermore, we believe that the proposed approach to control the remanent state by exploring driven (non-linear) dynamics can be applied to non-magnetic systems that are characterized by ground states. Sample fabrication The samples were fabricated using electron-beam lithography and lift-off processes. The double-dot structure has dimensions of 2 × 1 μm 2 with vertical contact length of 740 nm and thickness 48 nm. The separation between each pair is 1 μm and, therefore, dipole–dipole interactions between dot pairs can be neglected. To measure the resonance frequencies of the gyrotropic modes, the structures were fabricated on top of a shorted Cr (10 nm)/Au (300 nm) CPW with a 3-μm-wide signal line. Micromagnetic simulations Micromagnetic simulations [29] were performed using the standard Ni 80 Fe 20 parameters; an exchange stiffness constant of A =13 pJ m −1 , saturation magnetization Ms=8 × 10 5 A m −1 , gyromagnetic ratio γ =18.5 GHzper kOe, a dimensionless Gilbert constant α =0.01, cell size of 5 × 5 × 5 nm 3 and magnetocrystalline anisotropy was neglected. To avoid large computational times, the structural dimensions were reduced by half to 1 × 0.5 μm 2 rather than 2 × 1 μm 2 . The resonance frequencies of the system are obtained by sweeping the driving frequency from 300 to 900 MHz with a constant RF field amplitude of 1 Oe. The representative time evolution of the two magnetization components for both the polarity combinations ( p 1 p 2 =±1) are presented in Supplementary Fig. S2 . The calculated eigenfrequencies of the two modes are 530 ( p 1 p 2 =−1) and 580 MHz ( p 1 p 2 =+1). Qualitative analysis of the collective vortex modes was also performed. The details of this analysis are provided in Supplementary Methods . How to cite this article: Jain, S. et al. From chaos to selective ordering of vortex cores in interacting mesomagnets. Nat. Commun. 3:1330 doi: 10.1038/ncomms2331 (2012).